Octave-wide photonic band gap in three-dimensional plasmonic Bragg structures and limitations of radiative coupling Radiative coupling between oscillators is one of the most fundamental subjects of research in optics, where particularly a Bragg-type arrangement is of interest and has already been applied to atoms and excitons in quantum wells. Here we explore this arrangement in a plasmonic structure. We observe the emergence of an octave-wide photonic band gap in the optical regime. Compared with atomic or excitonic systems, the coupling efficiency of the particle plasmons utilized here is several orders of magnitude larger and widely tunable by changing the size and geometry of the plasmonic nanowires. We are thus able to explore the regime where the coupling distance is even limited by the large radiative decay rate of the oscillators. This Bragg-stacked coupling scheme will open a new route for future plasmonic applications such as far-field coupling to quantum emitters without quenching, plasmonic cavity structures and plasmonic distributed gain schemes for spasers. In optics, the coupling of oscillators, especially via their radiative fields, is one of the most fundamental subjects of research. A system consisting of oscillators that are periodically arranged at wavelength-scale distances in the propagation direction of light ( Fig. 1a ) shows similarities to passive photonic crystal structures [1] , where the propagating light is manipulated by a periodic refractive index modulation. However, incorporating oscillators into this type of structure leads to fundamentally different phenomena as the oscillators are mutually coupled via their radiation fields and therefore can exhibit collective resonances. 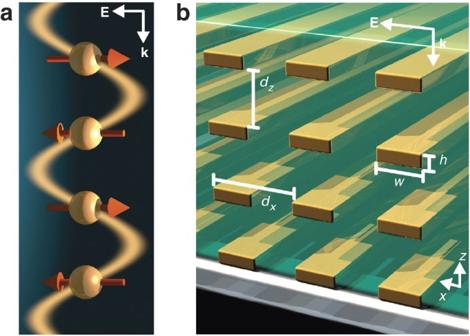Figure 1: Structure schematic. (a) Schematic of four radiatively coupled resonant oscillators. Considering retardation is crucial because of interparticle distances on the order of the wavelength. (b) Schematic of a Bragg-stacked plasmonic structure embedded into a dielectric spacer material with refractive indexnSp. Gold nanowires withw=180 nm andh=20 nm are arranged at a lateral periodicitydx=360 nm and vertical distancedz=260 nm.dxis chosen such that lateral near-field coupling as well as higher diffraction orders are negligible. Figure 1: Structure schematic. ( a ) Schematic of four radiatively coupled resonant oscillators. Considering retardation is crucial because of interparticle distances on the order of the wavelength. ( b ) Schematic of a Bragg-stacked plasmonic structure embedded into a dielectric spacer material with refractive index n Sp . Gold nanowires with w =180 nm and h =20 nm are arranged at a lateral periodicity d x =360 nm and vertical distance d z =260 nm. d x is chosen such that lateral near-field coupling as well as higher diffraction orders are negligible. Full size image This type of coupled system has previously been considered in several fields of optics: in semiconductor physics, radiative coupling of excitons in quantum wells [2] , [3] , [4] , [5] , [6] , [7] , [8] at Bragg distance leads to superradiant coupling effects and a photonic band gap (PBG). For 100 coupled quantum wells, the formation of a PBG of 5 meV width has been demonstrated [6] . Likewise, atoms arranged in an optical lattice can give rise to PBGs of several megahertz to gigahertz linewidth [9] , [10] , [11] , [12] . Here we transfer this concept to plasmonics, where up to now, mostly laterally coupled, planar structures have been studied [13] , [14] , [15] , [16] , [17] , [18] , [19] , [20] , [21] , [22] , [23] , [24] , [25] , [26] , and only little work in three-dimensional, stacked geometries has been performed [14] , [27] . A stacked arrangement is advantageous for several reasons. First, the oscillators are excited with a phase retardation and thus the spatial forward–backward symmetry is broken. Eigenmodes which are dark in planar geometry can become bright in a stacked geometry. Second, the dipole emission patterns of the oscillators are aligned along the interparticle axis, which substantially enhances the interaction strength. We stack plasmonic oscillators with a particle plasmon resonance (PPR) at wavelength λ PPR in Bragg fashion. Figure 1b shows a schematic of the structure, which consists of vertically stacked gold nanowires separated by a dielectric spacer layer. The structure is illuminated from above with light polarized perpendicular to the nanowires. We observe an octave-wide PBG at optical frequencies, characterized by a broad region of high reflectance with simultaneously weak absorbance. Furthermore, we identify the limitation of radiative coupling due to the extremely fast decay of the resonant plasmonic oscillators. Unlike in atomic or semiconductor systems, we are able to continuously tune the resonance frequency and oscillator strength of our classical oscillators over a range of nearly one order of magnitude and hence are able to engineer their properties easily. 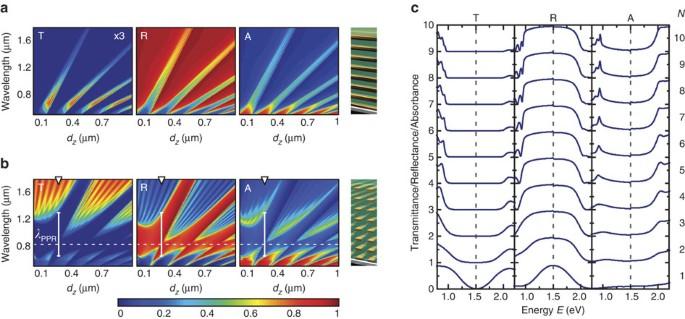Figure 2: Calculation results. (a) Colour-coded calculated transmittance, reflectance, and absorbance spectra for eight stacked 20-nm-thick continuous Au layers. The spacer thicknessdzis varied to the right. Transmittance is scaled by a factor of three for clarity. (b) Colour-coded calculated transmittance, reflectance, and absorbance spectra for an eight-layer plasmonic nanowire stack withλPPR=820 nm. Bragg spacing is indicated by a white arrow at the top of the graph. White solid lines indicate the width of the stop band at Bragg distance. The white dashed line indicates the single layer PPR wavelengthλPPR. The images on the right schematically depict the considered structures. (c) Calculated transmittance, reflectance, and absorbance spectra for the Bragg-stacked (dz=260 nm) multilayer structures with increasing layer numberN. The single oscillator resonance frequency is indicated by a dashed grey line as a guide to the eye. Calculations of non-resonant and resonant structures To demonstrate the difference between a non-resonant structure showing only refractive index contrast and a resonant plasmonic structure, Figure 2 shows calculated spectra of an eight-layer metal-dielectric cavity and an eight-layer nanowire stack. Calculations are performed with a scattering matrix algorithm [28] , [29] . The optical properties of gold are taken from Johnson and Christy [30] . Figure 2: Calculation results. ( a ) Colour-coded calculated transmittance, reflectance, and absorbance spectra for eight stacked 20-nm-thick continuous Au layers. The spacer thickness d z is varied to the right. Transmittance is scaled by a factor of three for clarity. ( b ) Colour-coded calculated transmittance, reflectance, and absorbance spectra for an eight-layer plasmonic nanowire stack with λ PPR =820 nm. Bragg spacing is indicated by a white arrow at the top of the graph. White solid lines indicate the width of the stop band at Bragg distance. The white dashed line indicates the single layer PPR wavelength λ PPR . The images on the right schematically depict the considered structures. ( c ) Calculated transmittance, reflectance, and absorbance spectra for the Bragg-stacked ( d z =260 nm) multilayer structures with increasing layer number N . The single oscillator resonance frequency is indicated by a dashed grey line as a guide to the eye. Full size image The bare metal-dielectric stack ( Fig. 2a ) shows broad regions of high reflectance due to the continuous metal films. Transmittance is only possible at the Fabry–Pérot (FP) modes, which are hybridized into seven branches as the structure consists of seven coupled cavities. In purely dielectric structures these hybridized modes would constitute the pass bands upon increasing layer number N . However, for metallic structures no pass bands emerge as absorbance increases significantly. Replacing the passive metallic layers by resonant metallic nanowires leads to substantial changes in the system, as is evident from Figure 2b . First, the off-resonant behaviour changes: the metal film exhibits a high reflectivity over a broad spectral region, consequently showing high reflectance and no transmittance. In contrast, far away from the PPR wavelength, the nanowire structure shows higher transmittance and low reflectance. Second, the incorporation of the PPR oscillators qualitatively changes the response of the system as the interaction of FP and PPR modes leads to the formation of coupled PPR-FP modes [27] . This opens up new possibilities to tune the response of the system. A situation of particular interest occurs whenever the vertical spacing matches a multiple of the single oscillator wavelength, that is, with an integer number M . At these points, the Bragg criterion for the PPR wavelength is fulfilled and the oscillator phases are adjusted such that their emitted fields interfere destructively in the forward direction and constructively in the backward direction. Consequently, the system exhibits high reflectance and low transmittance. As the coupled PPR–FP modes which spectrally match the single oscillator wavelength exhibit a nearly vanishing linewidth due to the spatially matched arrangement of the oscillators [27] , the spectral width of this region of high reflectance, low transmittance, and almost no absorbance (indicated by white solid lines in Fig. 2b ) is very broad. To investigate the influence of increasing oscillator number N in our plasmonic system, Figure 2c shows calculated transmittance, reflectance, and absorbance for one to ten nanowire layers stacked at Bragg distance. An increase of the width of the high-reflectance region can be observed. Beyond this, the spectral shape changes from a Lorentzian-like to a rectangular PBG-like shape. The high reflectance is accompanied by very low absorbance, which is only significant at the borders of the gap. The spectral width of 1 eV is remarkable, as it spans almost one octave. The reason for the emergence of this exceptionally broad PBG is the efficient coupling of the PPRs to the light field and hence their large spectral width compared with excitonic structures. This will be discussed in detail below. Experiment We fabricated a sample that consists of four layers stacked at Bragg distance by using an electron-beam lithography multilayer process [27] , [31] . 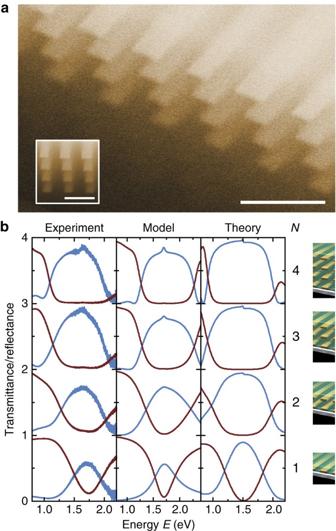Figure 3: Experimental data and comparison. (a) Scanning electron micrograph of a four-layer plasmonic Bragg structure. To reveal the three-dimensional arrangement, the images show a groove cut by a focused ion beam. All scale bars are 500 nm. (b) Left: experimental transmittance (red) and reflectance (blue) spectra for one to four layers. Middle: spectra calculated using an analytical coupling model7. The oscillator parameters extracted from the single-layer experimental data were used as calculation input. Right: scattering matrix calculation. The small peak in reflectance at 1.5 eV is a remainder of the coupled PPR–FP mode whose linewidth almost vanishes at Bragg distance. The images on the right schematically depict the structure. A scanning electron micrograph of the sample is shown in Figure 3a . Transmittance as well as reflectance spectra were recorded in a Fourier-transform infrared microscope after the completion of each layer. The evolution of the spectra with increasing layer numbers is shown in Figure 3b experimentally as well as theoretically, using an analytical coupling model [7] (see Methods ), and furthermore, a rigorous scattering matrix approach. The transformation of the spectral shape from a Lorentzian lineshape in the one-layer case to a rectangular band-gap-type lineshape for a Bragg multilayer stack is pronouncedly observable. The PBG in the four-layer structure, extracted from the reflectance measurement exhibits a spectral width of 815 meV, whereas the single PPR width is only 530 meV. Both of these values are slightly below the calculated values of 1,025 and 640 meV, respectively. In the gap region, the structure exhibits a very high reflectivity of around 80% experimentally, whereas the calculated reflectance is at almost 100%. Deviations between theory and experiment predominantly originate from fabrication imperfections, and the measurement technique using a high-NA Cassegrain objective. Figure 3: Experimental data and comparison. ( a ) Scanning electron micrograph of a four-layer plasmonic Bragg structure. To reveal the three-dimensional arrangement, the images show a groove cut by a focused ion beam. All scale bars are 500 nm. ( b ) Left: experimental transmittance (red) and reflectance (blue) spectra for one to four layers. Middle: spectra calculated using an analytical coupling model [7] . The oscillator parameters extracted from the single-layer experimental data were used as calculation input. Right: scattering matrix calculation. The small peak in reflectance at 1.5 eV is a remainder of the coupled PPR–FP mode whose linewidth almost vanishes at Bragg distance. The images on the right schematically depict the structure. Full size image Strikingly, we observe a broad, saturating PBG for already four layers, whereas in excitonic structures around 100 oscillators are necessary. As will be shown below, both the broad spectral width of the PGB and fast saturation arise from the large dipole moment of the PPR, which results in a radiative coupling strength exceeding that of a typical excitonic resonances by about four orders of magnitude. Additionally, this large coupling makes the emergence of a PBG in our plasmonic structures far more robust against nonradiative contributions to the linewidth. Analytical modelling To gain insight into the mechanisms that lead to the formation of broad PBGs, we study the influence of the coupling strength on band gap formation within a single oscillator model. If the lateral spacing between the nanowires within a layer is chosen such that near-field coupling can be neglected, each layer can be treated as a single, planar confined oscillator. Its optical response is then described by the effective susceptibility with resonance energy E PPR , and radiative and nonradiative linewidth Γ 0 and Γ, respectively. The radiative linewidth Γ 0 determines the oscillator strength and hence the coupling to the light field. In a multilayer structure, the oscillators couple via their radiation fields, which leads to N distinct modes. For semiconductor multi-quantum-well structures with narrow linewidths, it has been shown that in a Bragg arrangement only one superradiant mode couples to the light field and the collective response of the system resembles a single oscillator with N times enhanced radiative width [4] , [5] , [6] , [7] , [8] . The amplitude reflection coefficient is then given by: However, an unlimited growth of the linewidth N Γ 0 as implied by equation (2) is, of course, unphysical. It relies on the exact phase coherence of excitations in different layers. As the total linewidth determines the spectral width of the radiation field that contributes to the coupling of different layers, its spatial extent is limited by dephasing and can become smaller than the sample dimensions. Hence, the number of oscillators that can be efficiently coupled by the radiation field is limited by the dephasing length where equation (2) has been used in the latter equality. The condition Nd z < l d determines the number of layers that can be coupled in a Bragg geometry, resulting in For plasmonic oscillators, the radiative linewidth substantially exceeds the nonradiative contribution. The maximum number of coupled oscillator layers that yield approximately a Lorentzian lineshape can be estimated to be with a maximum total linewidth which is independent of the nonradiative losses. Stacking more layers changes the spectral shape of the reflectivity from a Lorentzian to the typical PGB shape. Its ultimate width can be calculated by considering an infinite structure and using a Kronig-Penney approach [32] which is achieved for a layer number of Oscillator strength tuning and limits of radiative coupling To further support the evidence for this radiation-limited coupling, we perform a set of scattering matrix calculations with decreased wire dimensions. As the oscillator strength depends on the number of electrons and thus on the volume of the wires, we tune the plasmonic oscillator strength by decreasing the width and height of the wires while the spectral position of the PPR is preserved. 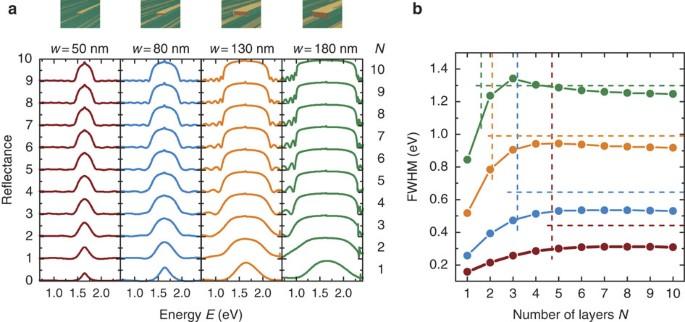Figure 4: Calculation results for different oscillator strengths. (a) Calculated reflectance spectra for increasing number of layersNof a Bragg stack with different wire geometries. The widths and heights of the wires are 50×4 (red), 80×6.8 (blue), 130×12.8 (orange) and 180×20 nm2(green). The images above schematically depict the structure. (b) FWHM extracted from the spectra in (a). Horizontal lines indicate the maximum band gap ΔEmax, vertical lines indicate the maximum number of layers that can be coupledNmax. The resulting reflectance spectra for four different geometries are shown in Figure 4a . The spectral linewidth extracted from these graphs is shown in Figure 4b . For all geometries, a saturation of the spectral width can be observed. The onset of saturation and the maximum width, however, depends on the wire geometry and hence the oscillator strength. One can calculate the maximum layer number N max as well as the maximum gap width Δ E max (Eq. 5) by extracting the values for Γ 0 and Γ from the single-layer spectra. These are indicated for the different geometries by vertical ( N max ) and horizontal (Δ E max ) lines in Figure 4b . The agreement is quite good for the large wires. For the smaller wires, Δ E max is overestimated, as the nonradiative contribution to the linewidth has not been taken into account in equation (5). Figure 4: Calculation results for different oscillator strengths. ( a ) Calculated reflectance spectra for increasing number of layers N of a Bragg stack with different wire geometries. The widths and heights of the wires are 50×4 (red), 80×6.8 (blue), 130×12.8 (orange) and 180×20 nm 2 (green). The images above schematically depict the structure. ( b ) FWHM extracted from the spectra in ( a ). Horizontal lines indicate the maximum band gap Δ E max , vertical lines indicate the maximum number of layers that can be coupled N max . Full size image These results demonstrate a fundamental limit for the radiative coupling of plasmons, as well as excitons, as follows: with increasing coupling strength, the width of the spectral response increases, while simultaneously the number of layers required to achieve the maximum stop band decreases. Only a limited number of oscillators can couple because of their fast decay rate. By using large plasmonic nanowires, which exhibit a very efficient coupling to the radiative field, we can realize a very broad PBG with only a small number of coupled oscillators. In conclusion, we have demonstrated that radiative coupling of multiple particle plasmonic oscillators at Bragg distance leads to the emergence of a very broad PBG of almost one octave at optical frequencies. The effortless tunability of the oscillators allows for a flexible and easy tailoring of very broad PBGs. Furthermore, this coupling scheme is potentially interesting for an efficient coupling of quantum emitters to the radiation field [33] . In the future, introducing phase jumps by defects in the Bragg stack could lead to high-Q localized modes [34] . Possible applications range from novel filters and resonant cavities [35] , [36] , [37] to plasmonic distributed gain [38] , low-loss metamaterials [39] and spaser concepts [40] . Calculation methods The calculated spectra of Figure 3b are obtained by a home-made code using the Fourier modal method [28] or scattering matrix method. This method is ideally suited for the description of structures that consist of several layers along the light propagation axis and are periodic in the other, lateral directions. The structure is divided into several layers. As the individual layers exhibit lateral periodicity in both directions, Maxwell's equations can be rigorously solved as an infinite-dimensional linear eigenvalue problem. Assuring proper convergence, the calculation is truncated yielding the scattering matrix of a single layer. Subsequently, all scattering matrices of the individual layers are combined by considering the appropriate boundary conditions. The calculation of metallodielectric structures within this method is hampered by the strong permittivity differences at the interfaces between metallic and dielectric components in the structure. To achieve good convergence, a high number of harmonics has to be considered. Alternatively, optimization methods such as adaptive spatial resolution and correct factorization rules allow for substantially decreased calculation times [29] . In the calculations, the structure is placed on top of a quartz substrate and each layer is embedded into a spacer layer . The top layer is also capped by a spacer layer to maintain a homogeneous environment. All dielectrics are assumed dispersion-free. For gold, the experimental values of Johnson and Christy [30] are used. For the calculations in Figure 4 , a Drude metal with a plasma frequency of 2,100 THz and a damping frequency of 21 THz is assumed for the gold structures. The analytical calculation of Figure 3b utilizes a single oscillator model. Within this model, the response of a single planar sheet is modelled by its effective two-dimensional susceptibility given by equation (1). For narrow resonances, the radiative linewidth can be approximated as for the frequency range of interest. However, for broad plasmonic resonances it is necessary to include this frequency dependence. In the multilayer structure, the layers are coupled by the propagating reflected and transmitted waves, and the overall response depends on the exact geometry of the structure via the phases accumulated by the propagating light waves. The overall transmission and reflection amplitudes for a system consisting of N oscillators are then obtained as [7] with the N -dimensional vector and N × N matrix containing the phases between the oscillators. The t ( E ) and r ( E ) exhibit N complex resonances. For a single layer, the reflection and transmission amplitudes given by the equations (6) and (7) are simplified to The reflectance | r ( E )| 2 is used to retrieve the values for Γ 0 and Γ from the FWHM and the maximum height of the calculated single-layer spectra in Figure 4 . For narrow resonances at exact Bragg distance, equation (7) gives the simplified result of equation (2). The coupling between two layers separated by a distance d is proportional to Inserting a complex energy the dephasing length is defined as the length at which the coupling is decreased by a factor of e . Fabrication and measurement methods Experimental realization of the multilayers is achieved using a multilayer electron-beam lithography technique. Each layer is exposed in a PMMA resist layer with subsequent development and evaporation of 2 nm Cr and 20 nm Au in an electron-gun evaporator. After lift-off, the structure is planarized using a spin-on-dielectric layer (Futurrex IC1-200). Its thickness is controlled using different solvent fractions, varying spin speed and multiple coating runs. The spectra are acquired using a commercial Fourier-transform infrared spectrometer (Bruker Vertex 80) with attached microscope (Bruker Hyperion). Light is polarized perpendicular to the wires. A ×15 Cassegrain objective with NA 0.4 is used to illuminate the sample, as well as to collect the transmitted and reflected light. Measurements for different spectral ranges are performed with a Si (1.3–2.2 eV) and an InGaAs photodiode (0.7–1.3 eV). Subsequently, the spectra are combined. Transmittance is measured with respect to the bare substrate. For the reflectance reference measurement, a 200-nm-thick Au mirror is used. How to cite this article: Taubert, R. et al . Octave-wide photonic band gap in three-dimensional plasmonic Bragg structures and limitations of radiative coupling. Nat. Commun. 3:691 doi: 10.1038/ncomms1694 (2012).